Highly modular bow-tie gene circuits with programmable dynamic behaviour Synthetic gene circuits often require extensive mutual optimization of their components for successful operation, while modular and programmable design platforms are rare. A possible solution lies in the ‘bow-tie’ architecture, which stipulates a focal component—a ‘knot’—uncoupling circuits’ inputs and outputs, simplifying component swapping, and introducing additional layer of control. Here we construct, in cultured human cells, synthetic bow-tie circuits that transduce microRNA inputs into protein outputs with independently programmable logical and dynamic behaviour. The latter is adjusted via two different knot configurations: a transcriptional activator causing the outputs to track input changes reversibly, and a recombinase-based cascade, converting transient inputs into permanent actuation. We characterize the circuits in HEK293 cells, confirming their modularity and scalability, and validate them using endogenous microRNA inputs in additional cell lines. This platform can be used for biotechnological and biomedical applications in vitro, in vivo and potentially in human therapy. Engineering of conditional gene expression systems in mammals and mammalian cells dates more than three decades back [1] , [2] . Their applications include cell lineage tracking [3] , tissue- or lineage-specific gene expression [4] , tissue engineering [5] , cell reprogramming [6] and cell type-specific therapy [7] . They usually require that gene expression can be controlled via endogenous inputs, such as tissue-specific promoters [8] , [9] , [10] , [11] , [12] , [13] , [14] or micro RNAs (miRNAs) [15] . These inputs can control a transgene directly or via a synthetic transactivator. Alternatively, irreversible gene knock-in/knock-out in a subset of cells in an organism [16] , [17] , [18] can be actuated via a site-specific recombinase such as Cre. These approaches have been successfully used to solve multiple problems; however, a universal framework that can be broadly applied to any kind of conditional actuation, is still lacking. Such a framework should include, first, a programmable module for integrating one or more endogenous signals to reach maximal selectivity and specificity. Second, a ‘plug-and-play’ component to determine the reversibility of the resulting action. Finally, the action itself should be customizable and scalable. Prior efforts in mammalian synthetic biology [19] , [20] , [21] have already achieved substantial progress towards establishing such framework [22] , [23] , [24] , [25] , [26] , [27] , [28] , [29] , [30] , [31] . However, most lines of work have focused on sensing and integration/computing components, while the construction of modular, programmable downstream actuation systems has not been sufficiently explored. Studies in systems biology uncovered an important natural architecture called ‘bow-tie’ [32] or ‘fan-in/fan-out’, which stipulates sensing and integration of multiple inputs into a single ‘knot’ that in turn distributes the result across multiple outputs. Unique features of this architecture are efficient use of resources and a trade-off between robustness and complexity. Importantly, the central knot position in the bow-tie architecture facilitates the addition and/or substitution of multiple inputs and outputs at the circuit periphery with minimal intervention in its core, resulting in higher modularity. Moreover, different ‘plug-and-play’ knot modules can define, in a predictable and programmable fashion, the precise manner in which the outputs are controlled. We reason that the bow-tie architecture is highly suitable for a general-purpose actuation framework and set out to demonstrate its proof-of-concept implementation in mammalian cells. Given the extensive work conducted previously on input integration modules, we decide to incorporate one of them into the network and focus major design thrust on the knot architecture and output distribution. Specifically, we use a synthetic module that selectively identifies a cell state by logically processing a number of up- and downregulated miRNA inputs [28] , [33] . As miRNAs are excellent selective cues for tissue- and disease-state identification [34] , [35] , [36] , [37] , [38] , [39] , [40] , [41] , a bow-tie system with miRNA integration module would be immediately applicable to selective actuation tasks. In this study we design, construct and validate large-scale integrated bow-tie circuits comprising two different knot configurations. In the first configuration, the knot contains a transactivator that controls a number of downstream components via an inducible promoter, resulting in a reversible gene induction. In the second configuration, the knot includes a transactivator, an inducible site-specific recombinase gene and an irreversible switch. We perform circuit optimization and characterization in HEK293 cells and demonstrate robust input–output mapping and the desired, knot-dependent dynamic behaviour. We then validate the circuits in additional cell lines using endogenously expressed miRNAs as inputs. We show that the different knot configurations perform consistently with expectation and that the outputs can be added or swapped in a modular manner. Circuit design and experimental set-up In the blueprint for the proof-of-concept bow-tie circuit, the fan-in component is a variant of an RNA interference (RNAi) classifier network [28] , logically integrating a number of over- and unexpressed miRNA inputs according to the logic formula ‘Output=miR-21 and not (miR-141) and not(miR-142) and not(miR-146a)’. Rather than converging on an output gene, the inputs fan into either of the two bow-tie knots: (i) a synthetic transactivator ( Fig. 1a ) or (ii) a transactivator controlling, via an inducible promoter, site-specific recombinase and a recombinase-triggered switch ( Fig. 1b ). The former implements reversible downstream actuation by concurrent induction of bow-tie outputs via an inducible promoter; the latter is used for irreversible actuation of bow-tie outputs furnished with recombinase-triggered switch elements. The circuit blueprint contains a number of unspecified components such as the transactivator, the inducible promoter, the recombinase and the recombinase-triggered switch. 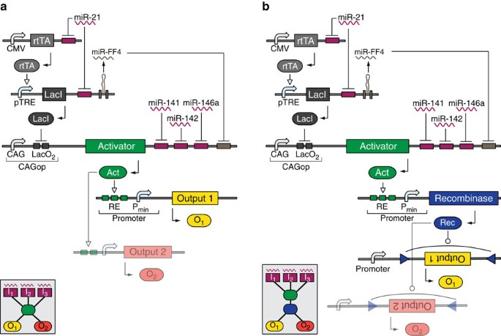Figure 1: Circuit blueprints of the bow-tie architecture. Both circuits are based on the same fan-in module that controls a synthetic transactivator by integrating miRNA inputs. The rtTA and LacI-based constructs sense ‘high’ miRNA input (miR-21), while targets in the 3′-untranslated region of the transactivator sense three ‘low’ miRNAs (miR-141, miR-142 and miR-146a). This arrangement triggers transactivator expression only in the presence of ‘high’ miR-21 and the absence of ‘low’ miR-141, miR-142 and miR-146a. DNA and RNA species are lumped together, with transcriptional control occurring on DNA level, while splicing and RNAi taking place on the RNA level. (a) Reversible knot configuration. The transactivator induces one or more outputs reversibly via an inducible promoter. (b) Irreversible knot configuration. The transactivator induces a recombinase that irreversibly modifies one or more outputs through an appropriate switch cassette. The insets show the high-level bow-tie wiring diagrams. Figure 1: Circuit blueprints of the bow-tie architecture. Both circuits are based on the same fan-in module that controls a synthetic transactivator by integrating miRNA inputs. The rtTA and LacI-based constructs sense ‘high’ miRNA input (miR-21), while targets in the 3′-untranslated region of the transactivator sense three ‘low’ miRNAs (miR-141, miR-142 and miR-146a). This arrangement triggers transactivator expression only in the presence of ‘high’ miR-21 and the absence of ‘low’ miR-141, miR-142 and miR-146a. DNA and RNA species are lumped together, with transcriptional control occurring on DNA level, while splicing and RNAi taking place on the RNA level. ( a ) Reversible knot configuration. The transactivator induces one or more outputs reversibly via an inducible promoter. ( b ) Irreversible knot configuration. The transactivator induces a recombinase that irreversibly modifies one or more outputs through an appropriate switch cassette. The insets show the high-level bow-tie wiring diagrams. Full size image We chose cultured human HEK293 cells as an experimental system for circuit development because (i) they represent a stringent testing environment due to high transcriptional activity and amplification of various ‘leakage’ phenomena, (ii) they lack miRNAs otherwise expressed in tumour cell lines and (iii) they can be transfected very efficiently. The latter feature allows exploring gene dosage required for robust circuit function by co-transfecting varying amounts of component-encoding plasmids (see below). Initial component selection We first developed the irreversible knot that requires efficient recombination combined with irreversible genetic switch, and tight control of the recombinase by the transactivator to prevent uncontrolled switching and resulting output expression. We tested iCre [42] , FlpO [43] and PhiC31o [43] enzymes with several irreversible switches, including PhiC31-inversion [44] , Cre-excision [45] , Cre-Flex [46] and FlpO-Flex [47] ( Fig. 2a , Supplementary Fig. 1a,b ). We measured switches’ response to increasing dose of constitutively expressed cognate recombinase and compared them with pre-recombined positive controls to estimate switching efficiency ( Supplementary Fig. 1c , Supplementary Table 1 , Supplementary Note 1 ). We found that all switches responded strongly to catalytic recombinase amounts. However, only Cre-Flex and FlpO-Flex showed high absolute response and efficiency and were retained for circuit development ( Fig. 2b ). 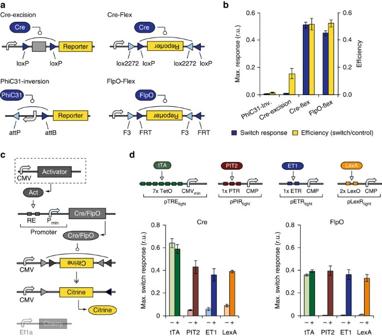Figure 2: Performance of irreversible recombinase switches. (a) Schematics of the four tested recombinase switches based on site-specific recombinases Cre, FlpO and PhiC31. The switch constructs undergo site-specific recombination in order to express constitutively driven reporter gene through various strategies (see alsoSupplementary Fig. 1). Triangles indicate recombinase recognition sites. (b) Maximal switch response (yellow bars) and corresponding efficiency (blue bars) of each switch. The efficiency is calculated as the ratio between recombinase-triggered reporter expression level and the expression level of pre-recombined control reporter in the presence of the same recombinase amount. Each bar represents mean±s.d. from three biological replicates measured 48 h after transfection using flow cytometry (see alsoSupplementary Fig. 1). Plasmid amounts are provided inSupplementary Table 1. (c) Schematics of the experimental set-up for testing regulated recombinase activity. A cytomegalovirus promoter-driven transactivator is co-transfected with a recombinase driven by an appropriate inducible promoter and a recombinase-triggered switch. (d) Top: activator–promoter combinations. Bottom: bar charts comparing the basal switch response (‘−’, no activator) and the maximal response observed with different transactivators (‘+’; see alsoSupplementary Fig. 2). Each bar represents mean±s.d. of three biological replicates measured 48 h after transfection using flow cytometry. Plasmid amounts are provided inSupplementary Table 2and quantitative readouts of the key samples inSupplementary Table 3. Figure 2: Performance of irreversible recombinase switches. ( a ) Schematics of the four tested recombinase switches based on site-specific recombinases Cre, FlpO and PhiC31. The switch constructs undergo site-specific recombination in order to express constitutively driven reporter gene through various strategies (see also Supplementary Fig. 1 ). Triangles indicate recombinase recognition sites. ( b ) Maximal switch response (yellow bars) and corresponding efficiency (blue bars) of each switch. The efficiency is calculated as the ratio between recombinase-triggered reporter expression level and the expression level of pre-recombined control reporter in the presence of the same recombinase amount. Each bar represents mean±s.d. from three biological replicates measured 48 h after transfection using flow cytometry (see also Supplementary Fig. 1 ). Plasmid amounts are provided in Supplementary Table 1 . ( c ) Schematics of the experimental set-up for testing regulated recombinase activity. A cytomegalovirus promoter-driven transactivator is co-transfected with a recombinase driven by an appropriate inducible promoter and a recombinase-triggered switch. ( d ) Top: activator–promoter combinations. Bottom: bar charts comparing the basal switch response (‘−’, no activator) and the maximal response observed with different transactivators (‘+’; see also Supplementary Fig. 2 ). Each bar represents mean±s.d. of three biological replicates measured 48 h after transfection using flow cytometry. 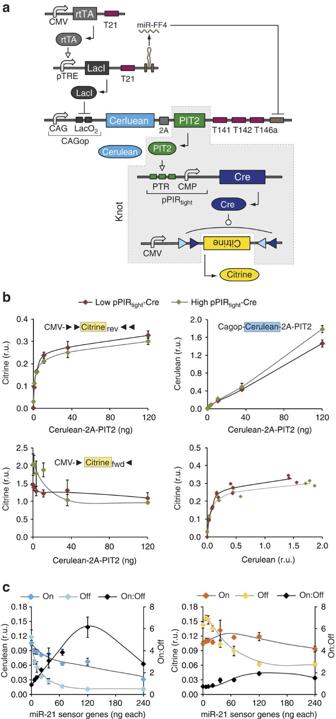Figure 3: First-iteration instantiation and characterization of irreversible bow-tie circuit. (a) Detailed circuit schematics. DNA and RNA species are lumped together, with transcriptional regulation and recombination taking place at the DNA level and splicing/RNAi at the RNA level. Different structural components of gene constructs are indicated. The knot components are shaded in grey. (b) Dose–response of CMV-CitrineCre-Flexto the amount of Cerulean-2A-PIT2. The Cerulean-2A-PIT2 cassette is co-transfected at varying levels with fixed amounts of pPIRtight-Cre and either CMV-CitrineCre-Flexor pre-recombined CMV-Citrine. Charts compare the dose–response of Cerulean and Citrine readouts generated in the presence of low (10 ng, red dots) or high (120 ng, green dots) amount of pPIRtight-Cre. Top row: responses measured with CMV-CitrineCre-Flex. Bottom left: Citrine readout from pre-recombined construct. Bottom right: Cerulean–Citrine transduction curves. The former three charts show mean±s.d. of biological triplicates with curves to serve as visual guides. The right-bottom chart shows individual triplicate measurements and a solid line is built by interpolation. (c) Dose–response of the On (+miR-21) and Off readouts (no miR-21) and the On:Off ratio to the amount of sensor-encoding plasmids. The dosage of both miR-21 sensor genes is changed simultaneously, while all the other components are kept constant. Separate readouts in On and Off states as well as the On:Off ratios are shown as indicated. Both charts show mean±s.d. of three biological replicates with manually drawn curves serving as visual guides. Error propagation rules were applied to calculate the s.d. of the ratio. Plasmid amounts used forb,care inSupplementary Table 4. Plasmid amounts are provided in Supplementary Table 2 and quantitative readouts of the key samples in Supplementary Table 3 . Full size image For inducible recombinase expression, we tested four different regulators namely the transactivators tTA-Advanced, PIT2 (Pip-p65) [48] , ET1 (MphR(A)-VP16) [49] and LexA-VP16 (ref. 50 ) in conjunction with their respective downstream promoters pTRE tight , pPIR tight , pETR tight and pLexR tight to drive Cre and FlpO expression. Apart from pTRE tight , the promoters were optimized for minimal leakage using specially designed core minimal promoter (Angelici et al ., submitted). Varying amounts of constitutively expressed transactivator were used to quantify dose–response and the efficiency was calculated using pre-recombined controls ( Fig. 2c,d , Supplementary Fig. 2 , Supplementary Tables 2 and 3 ). Between Cre and FlpO, Cre generated higher leakage in the absence of a transactivator and higher recombination efficiency. PIT2-, ET1- and LexA-driven switches shared low leakage, steep induction and certain decrease at high activator levels because of recombinase-induced inhibition of gene expression from already-recombined controls with high recombinase levels ( Supplementary Fig. 3 ). pTRE tight elicited full induction even in the absence of tTA, likely because of leaky CMV min in the promoter. As tight control of a recombinase is crucial, we chose PIT2/pPIR tight combination because of its superior dynamic range in conjunction with either Cre or FlpO recombinase and their respective Flex switches. Circuit optimization Component characterization allowed us to instantiate the unknown building blocks in order to create an irreversible bow-tie circuit (V1-Cre) by inserting the knot PIT2/pPIR tight -iCre/CMV-Citrine Cre-Flex downstream of the fan-in module. As fully assembled circuits contain large number of gene constructs and require multiplasmid cotransfection, we performed a number of tests to quantify the efficiency of multiple plasmid uptake in HEK293 cells. Our data showed that the efficiencies are reasonably high and permissive for our experimental set-up ( Supplementary Fig. 4 ). Next, we coupled PIT2 to the Cerulean fluorescent reporter via a 2A linker [51] in order to track fan-in module performance and placed the Cerulean-2A-PIT2-coding sequence under the control of the CAGop promoter, low-level miRNA inputs and auxiliary miR-FF4 ( Fig. 3a ). First, we recalibrated the core composition of the knot and optimized relative dosage of CAGop-Cerulean-2A-PIT2, pPIR tight -Cre and CMV-Citrine Cre-Flex constructs in order to ensure the desired linear ‘transfer function’ between Cerulean and Citrine reporters. Since we observed rapid saturation of the switch output, we tested whether small amounts of pPIR tight -Cre would maintain efficient switching while reducing the leakage in the absence of an activator. We found that dose–response of Citrine to Cerulean-2A-PIT2 was superior with low amount of pPIR-Cre, resulting in lower leakage of pPIR tight promoter and lower inhibition of pre-recombined product ( Fig. 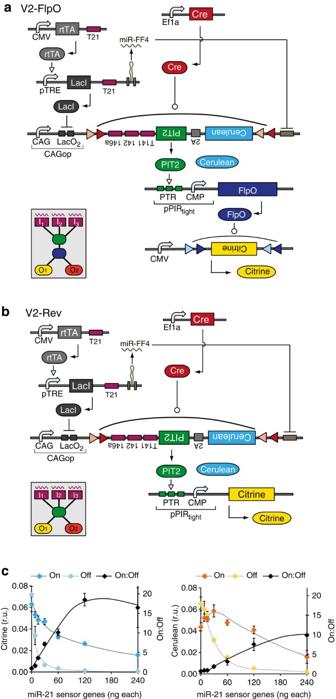Figure 4: Second-iteration bow-tie circuit instantiation and preliminary characterization. Detailed schematics of second-iteration circuits: irreversible V2-FlpO (a) and reversible V2-Rev (b). DNA and RNA species are lumped together, with transcriptional regulation and recombination taking place at the DNA level and splicing/RNAi at the RNA level. Different genetic building blocks are indicated. The insets show the high-level diagrams of the corresponding bow-tie architectures. (c) Dose–response of the On (+miR-21) and Off (no miR-21) readouts and the On:Off ratio to the amount of sensor-encoding plasmids in V2-FlpO. The amounts of miR-21 sensor genes are changed simultaneously, while all the other components are kept constant. Left and right charts show the changes in Cerulean and Citrine readouts, respectively. Both charts show mean±s.d. of three biological replicates with manually drawn curves serving as visual guides. Error propagation rules were applied to calculate the s.d. of the ratio. Plasmid amounts are provided inSupplementary Table 5. 3b , Supplementary Table 4a ). The results pointed to the optimal ratio of roughly 1:1:10 between knot genetic components. Figure 3: First-iteration instantiation and characterization of irreversible bow-tie circuit. ( a ) Detailed circuit schematics. DNA and RNA species are lumped together, with transcriptional regulation and recombination taking place at the DNA level and splicing/RNAi at the RNA level. Different structural components of gene constructs are indicated. The knot components are shaded in grey. ( b ) Dose–response of CMV-Citrine Cre-Flex to the amount of Cerulean-2A-PIT2. The Cerulean-2A-PIT2 cassette is co-transfected at varying levels with fixed amounts of pPIR tight -Cre and either CMV-Citrine Cre-Flex or pre-recombined CMV-Citrine. Charts compare the dose–response of Cerulean and Citrine readouts generated in the presence of low (10 ng, red dots) or high (120 ng, green dots) amount of pPIR tight -Cre. Top row: responses measured with CMV-Citrine Cre-Flex . Bottom left: Citrine readout from pre-recombined construct. Bottom right: Cerulean–Citrine transduction curves. The former three charts show mean±s.d. of biological triplicates with curves to serve as visual guides. The right-bottom chart shows individual triplicate measurements and a solid line is built by interpolation. ( c ) Dose–response of the On (+miR-21) and Off readouts (no miR-21) and the On:Off ratio to the amount of sensor-encoding plasmids. The dosage of both miR-21 sensor genes is changed simultaneously, while all the other components are kept constant. Separate readouts in On and Off states as well as the On:Off ratios are shown as indicated. Both charts show mean±s.d. of three biological replicates with manually drawn curves serving as visual guides. Error propagation rules were applied to calculate the s.d. of the ratio. Plasmid amounts used for b , c are in Supplementary Table 4 . Full size image Next, we placed the miR-21 sensor upstream of the knot in order to characterize circuit readouts under varying input conditions. We varied the dosage of sensor components and used miR-21 and negative control miRNA mimics to generate On and Off sensor states, respectively ( Fig. 3c , Supplementary Table 4b ). We found that the On:Off ratios, observed at the Cerulean/PIT2 level, deteriorated at the Citrine level because of amplification of the PIT2 leakage in the Off state. The best ratios were obtained with 120 ng of each sensor gene, resulting in overall dosage ratio of 10:10:1:1:10 in the cascade. The low On:Off ratios highlighted the importance of leakage suppression during signal transduction from the fan-in to the fan-out modules in the irreversible knot. In order to reduce this leakage, an approach was developed [52] whereby the miRNA sensor output itself is incorporated in a Flex switch in an inverted orientation. The orientation is restored by a constitutively expressed recombinase, resulting in a delay relative to the expression of sensor genes and leading to the accumulation of repressor species resulting in much lower Off state. We utilized this method, flanking the inverted Cerulean-2A-PIT2 by loxP and lox2272 sites as in Cre-Flex switch and providing EF1a-driven Cre in trans. FlpO replaced Cre in the irreversible knot resulting in PIT2/pPIR tight -FlpO/CMV-CIitrine FlpO-Flex knot configuration and in a circuit labelled V2-FlpO ( Fig. 4a ). We also constructed its reversible analogue, V2-Rev ( Fig. 4b ), where PIT2 directly controls output proteins via pPIR tight promoter. MiR-21 sensor characterization with V2-FlpO showed large improvement in both Cerulean and Citrine On:Off ratios ( Fig. 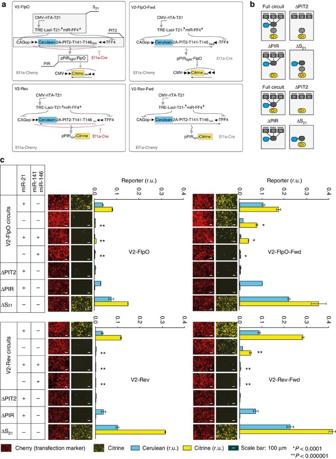Figure 5: Characterization of second-iteration circuits in microRNA profiling task. (a) Detailed circuits and their code names. Cerulean and Citrine readouts are highlighted. Shaded components with callouts in V2-FlpO diagram are removed one at a time in control experiments performed with this and other circuits. (b) Simplified diagrams showing complete circuits and various controls in the context of the bow-tie architecture corresponding to irreversible (top four) and reversible (bottom four) variants. (c) Experimental data. Each of the four circuits were transfected together with different miRNA input combinations as indicated in the tables on the left. The bar charts show normalized Cerulean and Citrine intensities as mean±s.d. from three independent biological replicates. Representative microscopy snapshots show the Citrine expression (yellow pseudocolour) and the transfection marker mCherry expression (red pseudocolour). Cerulean snapshots are not shown owing to very low Cerulean signal because of low plasmid dosage. Two-sided unpairedt-tests were performed for observed differences in Citrine in the Off-configuration samples (−/−, +/+, −/+) compared with the On configuration (+/−).Pvalues are indicated as follows: **P<0.000001, *P<0.0001. Transfection set-up is given inSupplementary Table 6and quantitative values inSupplementary Table 7. Representative flow cytometry plots and raw data are inSupplementary Fig. 5. 4c , Supplementary Table 5 ), as expected. Figure 4: Second-iteration bow-tie circuit instantiation and preliminary characterization. Detailed schematics of second-iteration circuits: irreversible V2-FlpO ( a ) and reversible V2-Rev ( b ). DNA and RNA species are lumped together, with transcriptional regulation and recombination taking place at the DNA level and splicing/RNAi at the RNA level. Different genetic building blocks are indicated. The insets show the high-level diagrams of the corresponding bow-tie architectures. ( c ) Dose–response of the On (+miR-21) and Off (no miR-21) readouts and the On:Off ratio to the amount of sensor-encoding plasmids in V2-FlpO. The amounts of miR-21 sensor genes are changed simultaneously, while all the other components are kept constant. Left and right charts show the changes in Cerulean and Citrine readouts, respectively. Both charts show mean±s.d. of three biological replicates with manually drawn curves serving as visual guides. Error propagation rules were applied to calculate the s.d. of the ratio. Plasmid amounts are provided in Supplementary Table 5 . Full size image Circuit performance In order to perform comprehensive circuits’ characterization, we first tested them in an miRNA profiling task, measuring their output at a fixed time point with different fan-in logical input combinations using miRNA mimics in HEK293 cells, whereby the input is either fully active (+) or completely inactive (−). We used miR-21 as the ‘high’ input and a mixture of miR-141 and miR-146a as a composite ‘low’ input, resulting in four possible combinations. The On state should only occur in the presence of miR-21 and in the absence of miR-141 and miR-146a (combination +/−), while the Off state is expected to occur in three other cases. In addition, we included two negative controls for each circuit: one without Cerulean-2A-PIT2 (ΔPIT2), to measure leakage from pPIR tight , another without PIR-driven construct (ΔPIR) to confirm the central role of this promoter; and a positive control without miR-21 sensor (ΔS 21 ) to determine maximal induction of the output. Furthermore, to quantify the effect of flexed PIT2 cassette, we assembled circuits containing pre-recombined, forward-facing Cerulean-2A-PIT2 genes denoted as V2-FlpO-Fwd and V2-Rev-Fwd and their corresponding controls ( Fig. 5a,b ). Figure 5: Characterization of second-iteration circuits in microRNA profiling task. ( a ) Detailed circuits and their code names. Cerulean and Citrine readouts are highlighted. Shaded components with callouts in V2-FlpO diagram are removed one at a time in control experiments performed with this and other circuits. ( b ) Simplified diagrams showing complete circuits and various controls in the context of the bow-tie architecture corresponding to irreversible (top four) and reversible (bottom four) variants. ( c ) Experimental data. Each of the four circuits were transfected together with different miRNA input combinations as indicated in the tables on the left. The bar charts show normalized Cerulean and Citrine intensities as mean±s.d. from three independent biological replicates. Representative microscopy snapshots show the Citrine expression (yellow pseudocolour) and the transfection marker mCherry expression (red pseudocolour). Cerulean snapshots are not shown owing to very low Cerulean signal because of low plasmid dosage. Two-sided unpaired t -tests were performed for observed differences in Citrine in the Off-configuration samples (−/−, +/+, −/+) compared with the On configuration (+/−). P values are indicated as follows: ** P <0.000001, * P <0.0001. 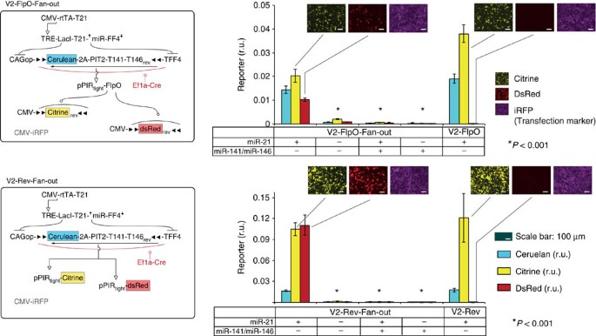Figure 6: Fan-in/Fan-out circuits. Left, schematics of the circuits V2-FlpO-fan-out and V2-Rev-fan-out. Right, corresponding quantitative data next to the single-output circuit V2-FlpO and V2-Rev used for comparison. Presence or absence of miRNA mimics is indicated on the bottom of the bar charts. Cerulean, Citrine and DsRed readouts are shown as mean±s.d. from three independent biological replicates; microscopy snapshots show Citrine (yellow pseudocolour), DsRed (red pseudocolour) and iRFP expression (magenta pseudocolour) and are given for On states (+/−) only. Two-sided unpairedt-tests were performed for observed differential output expression in On and Off states. Samples that havePvalues <0.001 in both Citrine and DsRed readouts are indicated. Transfection set-up is given inSupplementary Table 10, quantitative values inSupplementary Table 11and scatter plots as well as raw data are inSupplementary Fig. 8. 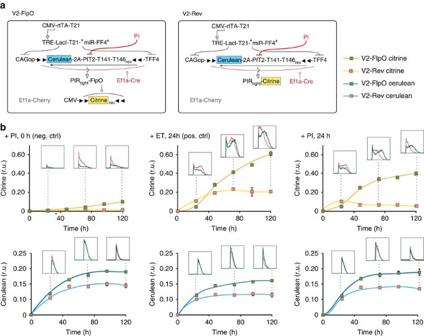Figure 7: Dynamic circuit behaviour. (a) Circuit schematics. PI inhibition of PIT2 is shown in red. (b) Time course charts of Cerulean and Citrine circuit readouts, normalized to transfection control. In each chart, mean±s.d. from three independent biological replicates are shown apart from a few points where a duplicate was measured (seeSupplementary Fig. 9). Each chart compares the behaviour of reversible (V2-Rev) and irreversible (V2-FlpO) knot architectures when PI is added at time zero (+PI, 0 h), a non-cognate antibiotic is added after 24 h (+ET, 24 h) or PI is added after 24 h (+PI, 24 h). Flow cytometry histograms gated for positive cells are shown for selected time points as indicated by dotted lines. Equal number of total events and equal axis scale are used to build the histograms, making them directly comparable. Transfection set-up is given inSupplementary Table 12, quantitative values inSupplementary Table 13and flow cytometry scatter plots inSupplementary Fig. 9. Transfection set-up is given in Supplementary Table 6 and quantitative values in Supplementary Table 7 . Representative flow cytometry plots and raw data are in Supplementary Fig. 5 . Full size image Comparison of the V2-FlpO and V2-Rev to their pre-recombined counterparts V2-FlpO-Fwd and V2-Rev-Fwd, respectively, showed a substantial improvement in the worst-case Off state (miR-21 minus miR-141-146a minus ) in both Cerulean and Citrine signals, consistent with observations in Figs 3 and 4 . In fact, Cerulean levels in many Off states in these circuits were indistinguishable from Cerulean autofluorescence measured with the control ΔPIT2 ( Fig. 5c , Supplementary Fig. 5 , Supplementary Tables 6 and 7 ). The On:Off ratio of the Citrine output improved from twofold in V2-FlpO-Fwd to 12- to 26-fold in the V2-FlpO circuit, and from sevenfold to 127-fold between the V2-Rev-Fwd and V2-Rev circuits. As a trade-off, we observed a reduction of ~50% in the On state. This decrease is mirrored by similar reduction in the output of ΔS 21 controls, suggesting that it is due to imperfect inversion of the Cerulean-2A-PIT2 by Ef1a-Cre and a minor contribution from the reduction in cotransfection efficiency ( Supplementary Fig. 4 ). Among the controls, ΔPIT2 circuits showed very low Citrine expression, confirming that the major cause of signal deterioration in the knot is insufficient repression of the Cerulean-2A-PIT2. However, additional design effort may be required to reduce the leakage of pPIR tight to zero. The performance of ΔPIR circuits conclusively illustrated the decoupling between the fan-in and fan-out modules: Cerulean levels were the same as in the complete circuits, while Citrine was virtually undetectable. Finally, for full comparison we performed similar measurements with first-iteration circuits and observed very similar performance to forward-facing V2 controls ( Supplementary Figs 6 and 7 , Supplementary Tables 8 and 9 ). Using the leakage-reducing strategy with expression-delayed, flexed Cerulean-2A-PIT2 construct in conjunction with the extensive optimization of the remaining components resulted in robust system performance. We proceeded to establish the complete bow-tie architecture with the knot controlling multiple outputs. We added output constructs expressing red-fluorescent protein (pPIR tight -DsRed and CMV-DsRed FlpO-Flex ), generating V2-Rev-fan-out and V2-FlpO-fan-out circuits, each controlling two independent outputs. The levels of Citrine and DsRed outputs were measured 48 h after transfection in an miRNA profiling task in a manner similar to single-output circuits. Since we used an iRFP (infrared fluorescent protein) as a transfection control in these experiments, we also re-measured V2-Rev and V2-FlpO circuits for comparison. Both V2-Rev-fan-out and V2-FlpO-fan-out circuits could simultaneously control both outputs in a manner consistent with miRNA input combinations ( Fig. 6 , Supplementary Fig. 8 , Supplementary Tables 10 and 11 ). Figure 6: Fan-in/Fan-out circuits. Left, schematics of the circuits V2-FlpO-fan-out and V2-Rev-fan-out. Right, corresponding quantitative data next to the single-output circuit V2-FlpO and V2-Rev used for comparison. Presence or absence of miRNA mimics is indicated on the bottom of the bar charts. Cerulean, Citrine and DsRed readouts are shown as mean±s.d. from three independent biological replicates; microscopy snapshots show Citrine (yellow pseudocolour), DsRed (red pseudocolour) and iRFP expression (magenta pseudocolour) and are given for On states (+/−) only. Two-sided unpaired t -tests were performed for observed differential output expression in On and Off states. Samples that have P values <0.001 in both Citrine and DsRed readouts are indicated. Transfection set-up is given in Supplementary Table 10 , quantitative values in Supplementary Table 11 and scatter plots as well as raw data are in Supplementary Fig. 8 . Full size image Dynamic circuit behaviour Next, we analysed circuit dynamics in order to confirm the reversible and irreversible nature of the two knot configurations in V2-Rev and V2-FlpO circuits, respectively. The output is expected to track the result of integration in the fan-in module in a reversible knot, while reflecting past fan-in history with the irreversible one. In the latter, removal of PIT2 signalling should not result in concomitant output decrease. The most direct way to illustrate this distinction is by directly inactivating PIT2 with the antibiotic Pristinamycin IA (PI) [53] ( Fig. 7a ). We applied PI at time zero and 24 h post transfection, while a control measurement was performed by adding a non-cognate antibiotic Erythromycin (ET) at 24 h. We measured Cerulean and Citrine levels every 24 h for 5 days using flow cytometry. The miRNA profile was established at the onset of the experiment to produce an On state in the fan-in module by transfecting miR-21 mimic. Figure 7: Dynamic circuit behaviour. ( a ) Circuit schematics. PI inhibition of PIT2 is shown in red. ( b ) Time course charts of Cerulean and Citrine circuit readouts, normalized to transfection control. In each chart, mean±s.d. from three independent biological replicates are shown apart from a few points where a duplicate was measured (see Supplementary Fig. 9 ). Each chart compares the behaviour of reversible (V2-Rev) and irreversible (V2-FlpO) knot architectures when PI is added at time zero (+PI, 0 h), a non-cognate antibiotic is added after 24 h (+ET, 24 h) or PI is added after 24 h (+PI, 24 h). Flow cytometry histograms gated for positive cells are shown for selected time points as indicated by dotted lines. Equal number of total events and equal axis scale are used to build the histograms, making them directly comparable. Transfection set-up is given in Supplementary Table 12 , quantitative values in Supplementary Table 13 and flow cytometry scatter plots in Supplementary Fig. 9 . Full size image The data showed increasing and then stabilizing expression of Cerulean (normalized to constitutive transfection control) in both V2-FlpO and V2-Rev circuits independent of PI or ET ( Fig. 7b , bottom row, Supplementary Fig. 9 , Supplementary Tables 12 and 13 ). Note that since PI affects PIT2 post-translationally, Cerulean level does not reflect PIT2 activity once PI is introduced. On the other hand, dynamics of Citrine expression showed differential response and confirmed the anticipated distinction between the irreversible and the reversible knot configurations ( Fig. 7b , top row, Supplementary Fig. 9 , Supplementary Tables 12 and 13 ). When comparing the default On state of the circuits (+ET1, 24 h), we observed that V2-Rev circuit generated Citrine faster than the irreversible V2-FlpO, producing a higher Citrine output after 24 h. However, it reached quasi-steady state at about 48 h tracking the dynamics of Cerulean/PIT2, as expected. In the irreversible circuit, the Citrine output kept increasing despite stabilization in Cerulean/PIT2 levels, because of ongoing output inversion by FlpO. When PI was added 24 h after transfection, normalized Citrine output in the reversible configuration (V2-Rev) dropped immediately and kept decreasing in the next 4 days. On the contrary, in the irreversible configuration the output continued to increase, with a fast fivefold increase in the first 24 h following PI addition, and extra 70% increase over the following 72 h. Last, when PIT2 was inhibited at time zero, the evolution of transfection control-normalized Citrine signal showed the expected low, constant expression in the reversible case and certain leakage that increased with time in the irreversible configuration. The leakage is likely because of imperfect inhibition of PIT2 by PI as well as basal pPIR promoter activity, and it highlights the trade-offs inherent to genetic irreversibility because of its integrator-like response to past history. Introducing additional attenuation on recombinase expression in the Off state is a subject of future work. Sensing endogenous inputs Following extensive characterization in HEK293 cells, we examined whether the entire circuit can function in additional cell lines using endogenous miRNAs as inputs. We tested two cancer cell lines, HeLa and HuH-7, whose known miRNA profile is consistent with the On circuit output (miR-21 HIGH miR-141 LOW miR142 LOW miR-146 LOW , see Supplementary Fig. 10a ) and HEK293 cells that generate Off output in their natural state. The knockdown activities were confirmed with bidirectional reporters and found to be largely consistent, with the exception of intermediate miR-142 activity in HuH-7 cells ( Supplementary Fig. 10b ). As HeLa and HuH-7 have lower transfection efficiency, we utilized an earlier finding that placing SV40-iCre on the same backbone with the fan-in module output increases the inversion efficiency [52] . Thus, we combined SV40-iCre and Cerulean-2A-PIT2 cassettes on the same plasmid and adjusted upwards the amount of this construct to reach a higher On state. The circuits with this modification were dubbed V2.1-FlpO and V2.1-Rev ( Fig. 8a ). Both of them responded correctly to their endogenous miRNA inputs in HeLa, HuH-7 and HEK293 cells. We also measured a number of control circuits to validate our findings ( Fig. 8b , Supplementary Fig. 11 , Supplementary Tables 14 and 15 ). In the reversible case, the trends were fully consistent with expectation. The control ΔS 21 generated similar readouts to the On circuit in HeLa and HEK293, and a reduced readout in HuH-7 because of the weak endogenous expression of miR-142 (which acts on Cerulean-2A-PIT2). Both negative controls—‘Off’ and ΔPIT2—were very low, as expected. The complete circuit was On in HeLa and HuH-7 with Cerulean readout reduced relative to respective ΔS 21 readout and with Citrine output tracking the Cerulean. In the irreversible case, full circuit readouts were slightly higher compared with ΔS 21 , which is contrary to expectation but can be explained by experimental variability. More interestingly, the differences in Citrine output did not track respective differences in Cerulean in HeLa and HuH-7 cells in both the circuits and the controls. A simple explanation is that the recombination efficiency and/or speed are higher in HuH-7 cells than in HeLa; thus, the same amount of PIT2/Cre generates different outputs. Nevertheless, qualitative circuit function was consistent with expectation without requiring overly extensive optimization. Thus, our architecture is applicable to different scenarios and is not strictly limited to the chassis cell line where it has been originally established. 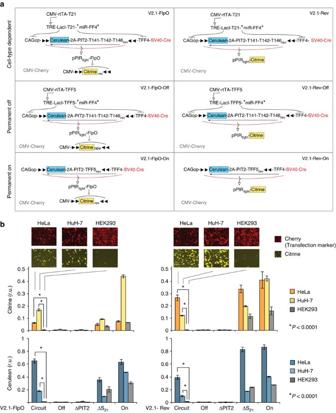Figure 8: Circuit operation in different cell lines. (a) Schematics of V2.1 circuits and corresponding controls specific to this set of experiments. The constitutive On and Off controls are used to measure the range of expression that is specific to each cell line. TFF5 is a control sequence that is not targeted by any known human miRNA. (b) Citrine (top) and Cerulean (bottom) readouts of the complete circuits and relevant controls compared across cell lines. Shown are mean±s.d. of three independent biological replicates measured 48 h after transfection using flow cytometry. Two-sided unpairedt-tests were performed to compare the differential output expression of the Circuit sample in HEK293 (Off state) compared with HeLa and HuH-7 (On states).Pvalues<0.0001 are indicated. Transfection set-up is given inSupplementary Table 14, quantitative values inSupplementary Table 15and scatter plots inSupplementary Fig. 11. Figure 8: Circuit operation in different cell lines. ( a ) Schematics of V2.1 circuits and corresponding controls specific to this set of experiments. The constitutive On and Off controls are used to measure the range of expression that is specific to each cell line. TFF5 is a control sequence that is not targeted by any known human miRNA. ( b ) Citrine (top) and Cerulean (bottom) readouts of the complete circuits and relevant controls compared across cell lines. Shown are mean±s.d. of three independent biological replicates measured 48 h after transfection using flow cytometry. Two-sided unpaired t -tests were performed to compare the differential output expression of the Circuit sample in HEK293 (Off state) compared with HeLa and HuH-7 (On states). P values<0.0001 are indicated. Transfection set-up is given in Supplementary Table 14 , quantitative values in Supplementary Table 15 and scatter plots in Supplementary Fig. 11 . Full size image The current report describes the bottom-up process of construction and characterization of a novel synthetic information-processing architecture inspired by the bow-tie concept. The design process was mostly guided by judicious application of current biological knowledge, and, given circuits’ complexity, relatively limited reliance on computational-aided design tools. Most causes of failure that we uncovered in measurements (for example, leaky promoters or low-efficiency recombination) would have been hard to predict using in silico simulations based on sequence alone. Nevertheless, the data we report here can be used to refine synthetic biology computational-aided design tools and broaden their applicability. Our data emphasize the importance of robust, leakage-free links between the building blocks. This is especially important in non-linear cascades of biological interactions where small signals can be greatly amplified. Extensive modifications that were made in the fan-in module, despite the fact that the module had been described previously, highlight the fact that integrating functional modules into larger networks is far from straightforward. One strategy is to employ signal restoration [54] ; however, the methodology for doing so in biological circuits is still under development. Our solution was to make individual components and modules behave in a highly ‘digital’ manner, in particular making sure that the ‘low’ or Off signals are very close to actual zero. For this purpose, we had to tune multiple knobs and use leakage-reducing strategies in inducible promoters and the fan-in module. Eventual demonstration of good performance characteristics suggests that once leakage is under control, a signal can travel through a long cascade without dissipation even in a coupled non-linear system. The longest chain of information flow in our circuits comprises miR-21 levels affecting rtTA/LacI/miR-FF4 concentrations, the latter controlling PIT2 activity in turn regulating FlpO levels that determine Citrine protein expression. We estimate that this could be one of the longest regulatory cascades implemented synthetically in a mammalian system. Robust architecture also allowed us to create some of the largest mammalian synthetic circuits, comprising up to seven separate genes. The bow-tie design is the key to scalability, as in the absence of a central knot, adding a second output to the classifier would require extensive optimization of five additional interactions (repression of the output by LacI, miR-FF4, miR-141, miR-142 and miR-146). Shifting the optimization burden to a reusable knot module allows facile swapping and adding of output genes. The uncoupling between inputs and outputs with the help of a modular knot offers a ‘plug-and-play’ approach to circuit construction. In particular, retroactive interactions between downstream and upstream modules in synthetic circuits have been identified as a possible challenge for composable, bottom-up design [55] . Our measurements demonstrated uncoupling between the upstream and downstream modules without detectable signs of retroactivity, therefore representing an attractive paradigm for circuit engineering. In the long term, a particularly interesting direction would be to use these circuits for selective cell fate reprogramming schemes that sense the initial cell state and only then trigger the reprogramming signals. In this case, the triggering should be irreversible because the initial state will likely disappear before the desired destination state is established. Circuits of this kind can also be used in cell-based therapies or tissue engineering to monitor current cell state and revert the state that has deviated from the ‘setpoint’ by continuous sensing of cell state-specific inputs. Such monitoring is best implemented by a reversible architecture. Plasmid construction Plasmids were constructed using standard cloning techniques. We used Escherichia coli DH5α as the cloning strain, cultured in LB Broth Miller Difco (BD) supplemented with appropriate antibiotics (Ampicillin, 100 μg ml −1 , Chloramphenicol, 25 μg ml −1 , Kanamycin, 50 μg ml −1 ). All enzymes were purchased from New England Biolabs (NEB). Phusion High-Fidelity DNA Polymerase (NEB) was used for standard fragment amplification (<6,000 bp) and LongAmp Taq DNA Polymerase (NEB) was used for amplification of large fragments (>6,000 bp). Single-stranded oligonucleotides used as primers or for annealing were provided by Microsynth or Sigma-Aldrich. Gene synthesis was performed by GenScript. Digestion products or PCR fragments were purified using the GenElute Gel Extraction Kit or Gen Elute PCR Clean Up Kit (both Sigma-Aldrich). All ligations were performed using T4 DNA Ligase (NEB) with individually adjusted incubation time and temperature, following transformation into chemically competent E. Coli DH5α and plating on LB Agar plates with appropriate antibiotics. Clones were analysed with colony PCR using Dream Taq Green PCR Master Mix (Thermo Scientific) or by test restriction after Miniprep purification of plasmids of individual clones using GenElute Plasmid Miniprep Kit (Sigma-Aldrich). All plasmids were sequenced by Microsynth. A short cloning procedure of each construct used in this work is described in the Supplementary Methods , with primers listed in Supplementary Table 16 . Plasmids used for transfection were purified from 100 to 400 ml cultures of E. coli DH5α grown overnight at 37 °C at ≈200 r.p.m. in LB Broth Miller Difco (BD) supplemented with appropriate antibiotic using the HiPure Plasmid Filter Maxi Kit (Invitrogen) or the PureYield Plasmid Midiprep Kit (Promega). After plasmid purification, an additional purification step was performed using the Endotoxin Removal Kit (Norgen Biotek Corporation). DNA amounts were quantified using Nanodrop (ND-2000) and integrity was verified with agarose gel electrophoresis. Cell culture HEK293 (293-H) cells were purchased from Life Technologies (Cat no. 11631–017) and cultured at 37 °C, 5% CO 2 in RPMI-1640 medium (Gibco, Life Technologies; Cat no. A10491-01), supplemented with 10% fetal bovine serum (FBS; Sigma-Aldrich; Cat no. F9665) and 1% Penicillin/Streptomycin Solution (Sigma-Aldrich; Cat no. P4333). Splitting was performed every 2–3 days at a cell density of 0.9–1.3 million cells per ml using 0.25% Trypsin-EDTA (Gibco, Life technologies; Cat no. 25200-072). HuH-7 cells were purchased from the Health Science Research Resources bank of the Japan Health Sciences Foundation (Cat no. JCRB0403, Lot no. 07152011) and cultured at 37 °C, 5% CO 2 in DMEM, low glucose, GlutaMAX (Life Technologies, Cat no. 21885-025), supplemented with 10% FBS (Sigma-Aldrich, Cat no. F9665 or Life Technologies, Cat no. 10270106) and 1% Penicillin/Streptomycin Solution (Sigma-Aldrich, Cat no. P4333). HeLa cells were purchased from ATCC (Cat no. CCL-2, Lot: 58930571) and cultured at 37 °C, 5% CO 2 in DMEM, high Glucose (Life Technologies, Cat no. 41966), supplemented with 10% FBS (Sigma-Aldrich, Cat no. F9665 or Life Technologies, Cat no. 10270106) and 1% Penicillin/Streptomycin Solution (Sigma-Aldrich, Cat no. P4333). Cultures were propagated for at most 2 months before being replaced by fresh cell stock. Transfections All transfections were performed using Lipofectamine 2000 Transfection Reagent (Life Technologies) in uncoated 24-well plates (Thermo Scientific Nunc). One day before transfection, cells were seeded into 500 μl medium per well at a cell densitiy of 7.5 × 10 4 for HEK293 and 6.5 × 10 4 for HeLa and HuH-7 per well. The medium was replaced with medium supplemented with Doxycycline hyclate (Fluka, Cat no. 44577) at a final concentration of 1 μg ml −1 shortly before transfection if required. Transfection was performed at 80–90% cell confluence and low passage number. The plasmids were mixed according to Supplementary Tables 1–9 and diluted with 50 μl Opti-MEM I Reduced Serum (Gibco, Life Technologies Cat no. 31985-962) per sample. If needed, miRNA mimics miR-21, miR-141, miR-146a and miR-Ctrl were added to the plasmid mix. All mimics were purchased from GE Healthcare. Exact miRNA mimic specifications can be found in Supplementary Table 17 . Lipofectamine 2000 was used in amounts of 1.5 μl ( Figs 2 and 3b , Supplementary Figs 1–3 ) or 1.8 μl ( Figs 3c and 4 , 5 , 6 , 7 , 8 , Supplementary Fig. 6 ) per sample and was mixed with 50 μl Opti-MEM. After 3 min incubation at room temperature, the diluted Lipofectamine was mixed with the diluted DNA sample. The mixture was incubated for 15 min at room temperature and added to the cells. Fluorescent microscopy Fluorescent images were generated 48 h after transfection by an inverted Fluorescent Microscope (Nikon Eclipse Ti) using a Fiber Illuminator (Nikon Intensilight C-HGFI), optimized optical filtersets (Semrock) and a Digital Camera System (Hammamatsu, ORCA R2). The filter sets contain a combination of excitation bandpass filter, emission bandpass filter and a dichroic filter for each individual fluorescent protein. We measured mCerulean, mCitrine, mCherry/DsRed and iRFP with the crosstalk minimized filter set CFP HC (HC 438/24, HC 483/32, BS 458), YFP HC (HC 500/24, HC 542/27, BS 520), TxRed HC (HC 624/40, HC 562/40, BS 593), Cy5.5-A (HC 655/40, HC 716/40, BS 685), respectively. We used an exposure time of 300 ms for circuit output mCitrine throughout all experiments and 2 s for DsRed output in Fan-out experiments in Fig. 6 . We used different exposure times for different transfection controls (Ef1a-Cherry, 20 ms, CMV-Cherry, 80 ms, CMV-iRFP, 2 s). The acquired images were uniformly contrast-enhanced for better visualization with the ImageJ software using LUT image intensity values 0–18,000 for mCitrine and mCherry, 0–35,000 for DsRed and 0–7,000 for iRFP, out of 65,000 (16-bit) intensity values. In Fig. 6 , LUTs of 1,500–5,000 were used for mCitrine. Flow cytometry All samples, apart from the samples in the time course experiment ( Fig. 7 ), were analysed 48 h after transfection by a BD LSR Fortessa cell analyser. The medium was removed and cells were incubated with 200 μl phenol-red free Trypsin (0.5% Trypsin-EDTA (Gibco, Life Technologies, Cat no. 15400-054) 1:2 diluted with phosphate-buffered saline (PBS; Gibco, Life Technologies, Cat no. 10010-56) for 3 min at 37 °C. Dispersed cells were transferred to FACS tubes (Life Systems Design, Cat no. 02-1412-000) and kept on ice. We used reporter-specific combinations of excitation lasers and emission filters for the detection of the different fluorescent reporters. For mCherry and DsRed, we used a 561-nm excitation laser, a 600-nm longpass filter and a 610/20-emission filter. For mCitrine and EGFP, we used a 488-nm Laser, 505-nm Longpass filter and a 542/27-nm emission filter. For mCerulean we used a 445-nm Laser and a 473/10 nm emission filter. For iRFP, we used a 640-nm Laser and a 710/50-emission filter ( Fig. 6 ) or 780/60 emission filter ( Supplementary Fig. 4 ). We used consistent PMT throughout all experiments. For circuit relevant measurement, this was a PMT of 220 V for both mCitrine and mCherry and a PMT of 460 V for mCerulean. SPHERO RainBow Calibration particles (Cat no. 559123, BD) and Align Flow Cytometry beads (Cat no. A16500, Life Technologies) were used to ensure constant device performance and PMTs were occasionally adjusted to compensate for changes in machine configuration. The PMT values of all experiments are indicated in the corresponding description of the experimental set-up. Data analysis All flow cytometry data were analysed using FlowJo software. Compensation of minor crosstalk (<1.2%) of mCherry into the 445–473/10 nm channel, of DsRed into the 445–473/10 nm and 488–542/27 nm channel, and of mCitrine into the 445–473/10 nm and in 561–610/20 nm channel was performed if necessary using FlowJo compensation matrix. The matrix coefficients were derived from the slopes of the best fit of the linear regressions of each single-colour control into each channel, calculated in MATLAB using exported single-colour control data. In order to perform adequate data analysis and interpretation of our results, we performed extensive investigation of transfection and expression characteristics in HEK293 ( Supplementary Fig. 12 , Supplementary Note 2 ). The values in the various charts, shown in relative expression units (r.u. ), are calculated as follows. (i) Live cells are gated based on their forward and side scatter readouts. (ii) Within this gate, cells that are positive in a given fluorophore are gated using fluorophore-negative, transfection marker-positive single-colour control such that 99.9% of cells in this single-colour control sample fall outside of the selected gate. See also gating strategy in Supplementary Fig. 13 . (iii) For each positive cell population in a given channel, the mean value of the fluorescent intensity is calculated and multiplied by the frequency of the positive cells. This value is used as a measure for the total reporter signal in a sample. The total reporter signal of an output was normalized with the total signal of the transfection control fluorophore to counterbalance possible transfection variation. The procedure can be summed in the following formula: Reporter intensity of a sample in r.u.=[mean (Reporter in Reporter+cells) × Frequency (Reporter+cells)]/[mean (Transfection Marker in Transfection Marker+cells) × frequency (Transfection Marker+cells)]. Data points in figures are shown as mean±s.d. of three independent biological samples. Error propagation rules were applied to calculate the s.d. of On/Off ratios. A two-sided unpaired homoscedastic t -test was performed on samples where On:Off ratios were measured. P values are indicated in figures as required. Histograms in Fig. 7 were created as follows: a representative sample was selected from three biological triplicates. Samples were compensated as described and gated for equal amounts of living cells. Histograms were built using gated fluorophore-positive cells in each channel and overlaid in FlowJo. For flow cytometry scatter plots of Supplementary Figs 5, 7–9 and 11 , one representative sample was selected from three biological replicates and gated for equal number of live cells. Owing to smaller sample size of HuH-7, some samples were concatenated to produce scatter plots with equal amounts of living cells. Long-term time course measurements The transfection procedure was performed using six-well plates (NUNC). One day before transfection, 2.5 × 10 5 HEK293 cells were seeded. Before transfection, the medium was replaced with 2,500 μl medium supplemented with 1 μg ml −1 Doxycycline hyclate per well. Transfection was performed as described above with DNA amounts and reagents scaled-up fivefold ( Supplementary Table 8 ). Each plasmid mixture was transfected in three groups of triplicates. The first triplicate was supplemented with antibiotics Pristinamycin IA (PI) (Molcan Corporation) right before transfection, the second triplicate was supplemented with PI 24 h post transfection and the last triplicate with or ET (Sigma-Aldrich) at a concentration of 1 μg ml −1 . To avoid confluency, cells were split in 1:3 ratio at 24 h, a sample taken to flow cytometry for a 24-h time point, and the rest of the cells distributed over four 24-well plate wells (with appropriate antibiotics replenished). One of the wells was measured with flow cytometry at 48 h. The cells in the remaining three wells were trypsinized and mixed at 72 h. A sample was measured to provide a 72 h time point, and the rest split 1:3 and replated into separate wells. The cells in these wells were measured with flow cytometry at 96 h and 120 h. How to cite this article: Prochazka, L. et al . Highly modular bow-tie gene circuits with programmable dynamic behaviour. Nat. Commun. 5:4729 doi: 10.1038/ncomms5729 (2014).